From protein sequence to dynamics and disorder with DynaMine Protein function and dynamics are closely related; however, accurate dynamics information is difficult to obtain. Here based on a carefully assembled data set derived from experimental data for proteins in solution, we quantify backbone dynamics properties on the amino-acid level and develop DynaMine—a fast, high-quality predictor of protein backbone dynamics. DynaMine uses only protein sequence information as input and shows great potential in distinguishing regions of different structural organization, such as folded domains, disordered linkers, molten globules and pre-structured binding motifs of different sizes. It also identifies disordered regions within proteins with an accuracy comparable to the most sophisticated existing predictors, without depending on prior disorder knowledge or three-dimensional structural information. DynaMine provides molecular biologists with an important new method that grasps the dynamical characteristics of any protein of interest, as we show here for human p53 and E1A from human adenovirus 5. Proteins derive their vast arrays of functions from the numerous interactions they have with each other and with other molecules in cells and organisms. These interactions are understood through knowledge of the three-dimensional (3D) structure of proteins in complex with their binding partner(s), an approach that is very successful and has led to many scientific breakthroughs. The dynamics of proteins, however, is also essential for their function, as exemplified by intrinsically disordered proteins (IDPs) [1] , [2] : they adopt an essential role in many biological processes and are implicated in pathogenic processes such as amyloid plaque formation in Alzheimer's. IDPs function as an ensemble of conformations and have no consistent 3D structure; their amino-acid residues will sample many different conformations, although they can still prefer certain conformations to others as determined by their sequence context [3] . Protein disorder is therefore related to dynamics; however, its identification and interpretation still pose a significant challenge. The key resource in the field, the DisProt database [4] , stores information on disordered regions through binary order/disorder (O/D) annotations on the amino-acid-residue level, which leads to the impression that a residue can behave only in two discrete ways. Such a clear distinction cannot be made; disorder is context-dependent, and many residues in non-globular proteins display a ‘dual personality’ [5] , where they exhibit a range of behaviours depending on environmental conditions. Within disorder, there are also distinctions to be made: a disordered residue can occur in many different conformational states and can occupy these with varying frequencies [6] , [7] , [8] . Another limitation is that the disordered regions in DisProt were often serendipitously observed and may therefore cover only a small and probably unrepresentative fraction of all disordered regions present in proteins. The >50 disorder predictors published to date [9] were almost all trained or tuned on DisProt annotations, and despite employing a large variety of computational principles and different subsets of carefully selected (structural) data, the resulting algorithms may not have the capacity to generalize beyond these data. Nuclear magnetic resonance (NMR) spectroscopy is the key technique to study dynamics and conformational states of proteins in solution at atomic resolution [10] , [11] . NMR-based case studies [12] , [13] , [14] have indicated that the level of conformational exchange of amino-acid residues is directly related to their dynamics, with fast dynamics indicating fast interchange between many (different) conformations. Information on fast local dynamics on the pico- to nano-second timescale can be obtained from NMR spin relaxation measurements; such fast motions are required for slower timescale dynamics such as conformational transitions [15] , [16] . These relaxation measurements entail, however, a considerable experimental effort, and the data are not routinely deposited in public archives. Much more accessible are the atomic-level chemical shifts, which are exquisitely sensitive to their environment. These chemical shifts give an averaged picture of local dynamics; however, they are abundantly available for a very diverse collection of proteins ranging from fully folded to disordered ones. To exploit this vast amount of data, we transform a carefully curated collection of chemical shifts for 2,015 of such proteins into a data set containing per-residue information on the fast movements of the protein backbone. This unique resource is directly rooted in experimental data closely connected to dynamics, gives a continuous and subtle picture of how amino-acid residues behave dynamically, and avoids the use of 3D structures [17] , [18] . It provides a statistical and quantitative view of the backbone dynamics properties for each amino acid that can be used to differentiate between the amino-acid tendencies to promote order or disorder. Using a linear regression approach, we construct DynaMine, an entirely novel method to accurately predict protein backbone dynamics directly from protein sequence. DynaMine identifies protein disorder as well as the most sophisticated existing predictors, but without using prior disorder information, instead depending on the underlying physical dynamics data. In doing so, it so firmly establishes the long anticipated link between dynamics of the polypeptide chain and structural disorder [19] , [20] . More importantly, it is the first direct predictor of dynamics from sequence, and we show through a range of case studies that it has great potential in distinguishing regions of different structural organization, such as folded domains, disordered linkers, structurally ambiguous molten globules and pre-structured binding motifs of different sizes. 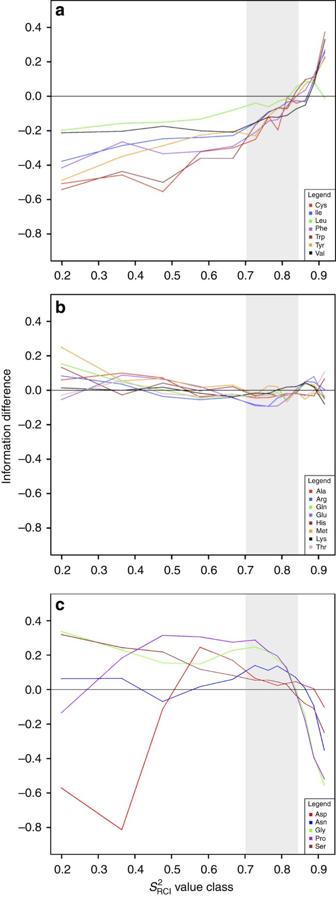Figure 1: Dynamics propensity per amino acid. Information difference per-based order class for amino acids that prefer order (a), are neutral (b) or prefer disorder (c). The grey zone indicates the intermediate dynamics zone between 0.70 and 0.85. Amino-acid backbone dynamics behaviour The core data set for the current work consists of backbone N-H S 2 order parameter ( ) values estimated from chemical shift values with the Random Coil Index (RCI) software [21] (see Methods) for 218,259 residues in 2,015 proteins from the BioMagResBank (BMRB) [22] (DS RCI-S2 , Table 1 ). Only those proteins were included that fulfil certain criteria regarding available chemical shift data, sample content and sample conditions (see Methods). S 2 order parameters represent how restricted the movement of an atomic bond vector is with respect to the molecular reference frame. A value of 1.0 signifies complete order (stable conformation), whereas a value of 0.0 means fully random bond vector movement (highly dynamic). The values capture motions from femtosecond up to nanosecond and possibly to higher timescales [21] and correspond with reasonable accuracy to experimentally determined S 2 order parameters ( ), a finding we reconfirmed (see Methods). Table 1 List of data sets and their content (also see Fig. 3 ). Full size table In an exploratory analysis, we filtered the DS RCI-S2 data and calculated for each amino acid their statistical propensities towards adopting particular values (see Methods); positive values indicate that an amino acid prefers to adopt that particular value (higher propensity), negative values that it does not. These propensities are shown per residue and value class in Fig. 1 , where we divided the amino acids into ordered (Cys, Phe, Ile, Leu, Val, Trp, Tyr) ( Fig. 1a ), neutral (Ala, Glu, Lys, Met, Gln, Arg, Thr) ( Fig. 1b ) and disordered (Asp, Gly, His, Asn, Pro, Ser) ( Fig. 1c ) types. Figure 1: Dynamics propensity per amino acid. Information difference per -based order class for amino acids that prefer order ( a ), are neutral ( b ) or prefer disorder ( c ). The grey zone indicates the intermediate dynamics zone between 0.70 and 0.85. Full size image The ordered residues show very similar propensities ( Fig. 1a ); they prefer backbone rigidity ( values >0.85) and have strong negative propensities for a dynamic backbone (low values). The one exception to this general trend is Leu, which has neutral propensity for very high values >0.9 and is less indisposed towards adopting highly dynamic states; this might indicate it is typically more involved in dynamic processes. The amino acids in this group exactly match prior knowledge about order-promoting amino acids [23] , [24] , [25] , which is related to hydrophobicity as was already established in the context of protein disorder [26] , [27] but are here quantified according to their backbone dynamics behaviour in proteins. The propensities for neutral residues remain close to zero ( Fig. 1b ). Some have slight propensities towards backbone rigidity: Ala, Arg, Gln, Glu and Lys have a preference for values of 0.85, whereas Thr has a slight tendency to adopt very high values. His and Met on the other hand have increased propensities for very low values, indicating their frequent occurrence in regions with a highly dynamic backbone. The residues we classified as disordered have neutral or negative propensities for a rigid backbone ( Fig. 1c ) and increased propensities for a more dynamic backbone ( values <0.8); Gly and Ser (the most disorder-promoting residues [23] , [25] ) maintain this preference for a highly dynamic backbone (very low values), whereas for Pro it drops to neutral. The profiles for Asp and Asn are interesting, as despite their small and hydrophilic sidechains they lack a strong propensity for highly dynamic states, possibly because of their capacity to form order-promoting sidechain to backbone hydrogen bonds. Asn has mostly neutral propensities, with a somewhat elevated propensity for values around 0.8. Asp, on the other hand, has a very low propensity for values <0.5, and an increased propensity for the 0.6–0.7 region. The typically negative charge of the carboxylic acid sidechain group in Asp could be responsible for this striking difference. These dynamics profiles show that differences between the classical order and disorder-promoting behaviour of amino acids can be quantified and identified based on the order parameters. Interestingly, the propensities for the ordered and disordered types switch side in the intermediate dynamics zone (grey zone in Fig. 1 ); this indicates the importance of this backbone dynamics region in determining amino-acid behaviour and highlights that it is not realistic to classify S 2 values, or disorder, in a binary sense: their spread is continuous, and applying a discrete cutoff imposes a naive meaning to the actual residue behaviour. Further improvements in the methodology to obtain dynamics information from chemical shifts, and inclusion of additional NMR data, will help to shed light on how each individual amino acid behaves with respect to disorder. It is however clear that the DS RCI-S2 data constitute a unique statistical resource on backbone dynamics in relation to individual amino acids. The linear backbone dynamics predictor DynaMine The DS RCI-S2 data set enabled us to develop DynaMine, a predictor of fast backbone dynamics from protein sequence only. We separated the DS RCI-S2 data set into two subsets: DS RCI-S2_NO_DP , with only sequences that have <90% sequence overlap with DisProt, and DS RCI-S2_DP , with sequences that have DisProt annotations ( Table 1 ). The DS RCI-S2_NO_DP data set was then used to train different linear regression models based on the size of the sequence window around the target amino acid (where a window size of, for example, 7 means that three amino acids on each side of the target amino acid are included). The performance of each predictor was evaluated by 10-fold cross-validation (see Methods). The linear correlation and Root Mean Squared Error (RMSE) ( Fig. 2a,b ), between the predicted S 2 order parameters ( ) and the actual values, improves as more of the amino-acid sequence context is taken into account. This is also evident from a parallel evaluation where the whole DS RCI-S2_NO_DP data set was used for training, all sequences in the DS RCI-S2_DP data set predicted and the resulting compared with the values ( Fig. 2c,d , blue). Although the improvements become less pronounced from a window size of 17 onwards, indicating that the residues influencing fast backbone dynamics are mostly nearby in the sequence, the window of 51 residues did give the best cross-validation results while still accounting for increased disorder in N- and C-terminal regions (see Methods). We selected this model for the final DynaMine implementation. 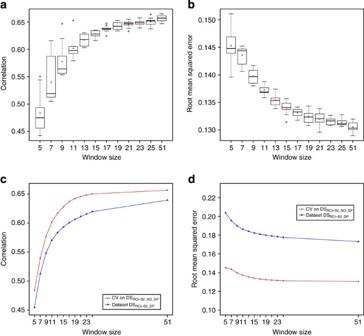Figure 2: Evaluation of DynaMine performance. Box plots, with bottom and top of the box representing the first (q1) and the third quartile (q3) of each distribution and the end of the whiskers atq1−1.5(q3-q1) andq3+1.5(q3-q1) of Pearson Correlation (a) and RMSE (b) of different 10-fold cross-validations of the linear regression model learnt from DSRCI-S2_NO_DPby varying the window sizew. Comparison of the Pearson Correlation (c) and RMSE (d) of different 10-fold cross-validations (mean values over the 10-folds) performed on DSRCI-S2_NO_DP(in red), with those of the predictions on the independent test set DSRCI_S2_DP(in blue). The predictions over the test data set DSRCI-S2_DPwere obtained from the linear regression model trained on DSRCI-S2_NO_DP. Figure 2: Evaluation of DynaMine performance. Box plots, with bottom and top of the box representing the first ( q 1 ) and the third quartile ( q 3 ) of each distribution and the end of the whiskers at q 1 −1.5( q 3- q 1 ) and q 3 +1.5( q 3- q 1 ) of Pearson Correlation ( a ) and RMSE ( b ) of different 10-fold cross-validations of the linear regression model learnt from DS RCI-S2_NO_DP by varying the window size w . Comparison of the Pearson Correlation ( c ) and RMSE ( d ) of different 10-fold cross-validations (mean values over the 10-folds) performed on DS RCI-S2_NO_DP (in red), with those of the predictions on the independent test set DS RCI_S2_DP (in blue). The predictions over the test data set DS RCI-S2_DP were obtained from the linear regression model trained on DS RCI-S2_NO_DP . Full size image DynaMine and traditional O/D prediction To explore the relation between dynamics and disorder, we examined the performance of the dynamics-related and values, as well as results from existing disorder predictors (IUPred [28] , PrDOS2 (ref. 29 ), RONN [30] , PONDR VSL2 (ref. 31 ), FoldIndex [32] and ESpritz [33] ), with respect to reproducing enhanced DisProt annotations for the sequences in the DS RCI-S2_DP set (see Methods and Fig. 3 ). The resulting receiver operating characteristic (ROC) curve clearly shows that the chemical shift-derived values ( Fig. 4a ) correlate very well with the DisProt annotations (Area Under the ROC Curve (AUC) of 0.916). The red curve almost always dominates; the chemical shift-derived data can identify disordered regions in the traditional binary O/D sense with the highest accuracy. Based on the ROC curve, a threshold of 0.795 for the values gives the best distinction between traditional O/D annotations; this corresponds well with the ‘crossover’ point of the per-amino-acid propensities from Fig. 1 . The black ROC curve shows the performance of DynaMine, which in this case was trained on DS RCI-S2_NO_DP (excluding DisProt sequences). The optimal threshold is 0.769 and matches the best threshold very closely. Of the existing disorder predictors, almost all of which have been trained on or are related to DisProt in some way, only the Espritz-NMR and PrDOS2 approaches perform better than DynaMine, which is completely independent of DisProt. In addition, these approaches often employ sophisticated prediction algorithms that incorporate complex information other than the simple amino-acid codes of the protein sequence used in DynaMine. ESpritz, for instance, is a consensus predictor based on complex bidirectional recurrent neural networks with input features including evolutionary information. PrDOS2 also takes into account evolutionary information and sequence conservation by means of BLAST profiles; as the winner of the CASP9 disorder-prediction competition, it can be considered as one of the most sophisticated existing disorder-prediction methods. 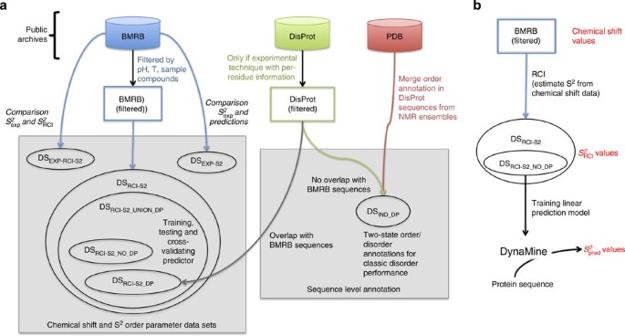Figure 3: Overview of the data sets and the method. An overview of the data sets used (a). The source public archives are given at the top; the left hand grey box shows the different data sets containing order parameter information and their relation to each other, the right hand grey box shows the sequence-level order/disorder annotations. The arrows from the public archive boxes give an overview of which data were used in which context. An overview of the relation between the DynaMine method, data sets and data values (in red) (b). Figure 3: Overview of the data sets and the method. An overview of the data sets used ( a ). The source public archives are given at the top; the left hand grey box shows the different data sets containing order parameter information and their relation to each other, the right hand grey box shows the sequence-level order/disorder annotations. The arrows from the public archive boxes give an overview of which data were used in which context. An overview of the relation between the DynaMine method, data sets and data values (in red) ( b ). 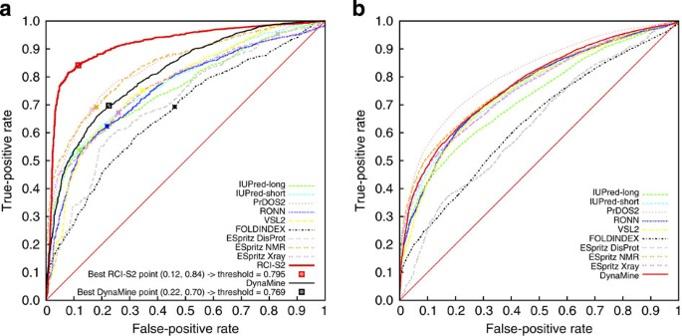Figure 4: Disorder-prediction performance. ROC curves for the prediction accuracy on data set DSRCI-S2_DP(a) and on the independent set of DisProt sequences DSIND_DPexcluding test set sequences in DSRCI-S2_DP(b). In the ROC curves for existing disorder predictors, the points indicate the best-performing threshold from the original papers. Full size image Figure 4: Disorder-prediction performance. ROC curves for the prediction accuracy on data set DS RCI-S2_DP ( a ) and on the independent set of DisProt sequences DS IND_DP excluding test set sequences in DS RCI-S2_DP ( b ). In the ROC curves for existing disorder predictors, the points indicate the best-performing threshold from the original papers. Full size image As the DS RCI-S2_DP set is small and biased towards proteins studied using NMR, we also examined the performance of and existing disorder predictors on a larger DisProt set (DS IND_DP ) of 241 sequences where experimental methods with residue-level resolution were used for O/D annotations (see Methods). The resulting ROC curve ( Fig. 4b ) shows that on this larger and more diverse set, the best-performing predictor is PrDOS2 (AUC of 0.811), followed by Espritz-NMR (AUC of 0.776). Moreover, DynaMine (AUC of 0.773) performs excellently, confirming the potential of the values in identifying traditional binary protein disorder annotations from a statistical backbone dynamics angle without incorporating prior information on disorder. This performance remains consistent across disordered fragments of different length (see Methods), although DynaMine especially excels at identifying short disordered fragments. In addition, the predictions go well beyond what hydrophobicity scales provide (see Methods). Biological relevance of the DynaMine predictions To qualitatively assess the relationship between the predicted backbone dynamics for proteins and their biological structure and function, we tested DynaMine on a set of well-studied proteins covering the full range of distinct structural and functional properties, including folded domains, molten globules and fully disordered regions that may fold upon binding. As is evident for the human cellular tumour antigen p53 ( Fig. 5a ), DynaMine can identify the boundaries of well-structured domains quite precisely: the DNA-binding domain (DBD) and the tetramerization domain are predicted to be ordered, whereas the linkers connecting these regions are highly dynamic. This ability to discriminate between domains and linkers is even more evident in case of the large, heterogeneous CREB-binding protein (CBP, Supplementary Fig. S1 and Supplementary Note 1 ). Within a structured region, as in p53 DBD, DynaMine is furthermore able to locate secondary structure elements; most secondary structure elements present in the free DBD correspond to peaks in the prediction pattern (see Supplementary Fig. S2 ). Secondary structure elements stabilized upon complex formation (p27, Supplementary Fig. S3 and Supplementary Note 1 ) also generally correspond to peaks in the prediction pattern. A range of additional case studies (human calpastatin, HIV Nef, and the Phd and PaaA2 antitoxins (see Supplementary Note 1 and Supplementary Figs S4–S7 )) further confirm that DynaMine is very good in distinguishing folded domains from disordered/highly dynamic linker regions, as well as in identifying flexible loop regions and secondary structure elements within globular domains. In case of HIV Nef ( Supplementary Fig. S5 ), the folded core of the protein is assembled from secondary structure elements quite distantly located from each other in the sequence; even then DynaMine predicts them as peaks within the more dynamic flexible loop regions. 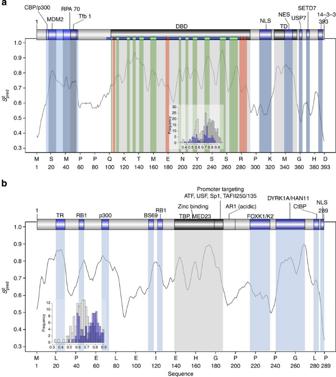Figure 5: DynaMine case studies. DynaMinevalues for the p53 human tumour suppressor (UniProt: P04637) (a) and the E1A from Human adenovirus 5 (UniProt: P03255) (b). The protein chain is in each case represented by a grey bar, with folded domains coloured black. For p53, binding regions corresponding to a subset of p53’s well-described interactions are presented by different shades of blue, and secondary structure is indicated in the DBD region (alpha helices—red, beta sheets—green). For E1A, well-described short linear motifs that mediate interactions with important factors of eukaryotic cell regulation are coloured light blue. The inset histograms show thevalue distribution colour-coded by the indicated domains (see alsoSupplementary Note 1andSupplementary Figs S2 and S8for full detail on histograms and annotation). Figure 5: DynaMine case studies. DynaMine values for the p53 human tumour suppressor (UniProt: P04637) ( a ) and the E1A from Human adenovirus 5 (UniProt: P03255) ( b ). The protein chain is in each case represented by a grey bar, with folded domains coloured black. For p53, binding regions corresponding to a subset of p53’s well-described interactions are presented by different shades of blue, and secondary structure is indicated in the DBD region (alpha helices—red, beta sheets—green). For E1A, well-described short linear motifs that mediate interactions with important factors of eukaryotic cell regulation are coloured light blue. The inset histograms show the value distribution colour-coded by the indicated domains (see also Supplementary Note 1 and Supplementary Figs S2 and S8 for full detail on histograms and annotation). Full size image The transactivation region (17–56) of p53 ( Fig. 5a ) is composed of different interaction motifs, each mediating the binding with multiple partners. This region is intrinsically disordered in the unbound form of p53 but folds up into alpha helices when binding to partners (for example, CBP/p300). DynaMine seems to recognize the inherent capability of these regions to fold up on binding, as it predicts scores intermediate between those predicted for folded domains and disordered regions. In CBP ( Supplementary Fig. S1 ), similarly intermediate values are observed for the NCBD molten globule domain, whereas for p27 ( Supplementary Fig. S3 ) the segment that folds up on complex formation with cyclin A/CDK2 has elevated values compared with the (disordered) remainder of the molecule. These observations indicate that the absolute values of the prediction might have meaning in the sense of domain stability. The prediction for adenovirus E1A, a host-regulatory viral hub protein, demonstrates the ability of our method to sense at least some interaction motifs ( Fig. 5b ). E1A is largely disordered with the exception of the central zinc-finger/promoter-targeting region; DynaMine renders the highest scores for this region. Plenty of known host-regulatory linear motifs are embedded in the disordered segments of its chain, and DynaMine identifies most of these interaction motifs by predicting definite peaks, indicating that they may have preformed structural elements. The linker/spacer regions are in contrast correctly predicted to be highly dynamic. The scores for known interaction sites thus separate well from those calculated for the remaining non-domain-disordered segments ( Fig. 5b , inset histogram and Supplementary Fig. S8 ), with the exception of residues at the C-terminal region and the end of the FOXK1/K2-binding region. Similarly, the distinct peaks predicted in p53 C-terminal-disordered region ( Fig. 5a ) correspond well to the short motifs previously described to fold up on binding to their partners. With this work, we demonstrate that statistical analysis of NMR data of proteins in solution can give quantitative insight into the relationship between amino-acid sequence and backbone dynamics. The DynaMine backbone dynamics predictor rests on S 2 order parameters directly estimated from experimental data content (NMR chemical shifts) and produces excellent results, despite the simple linear prediction methodology it uses. DynaMine is very fast and gives a continuous and subtle picture of how amino-acid residues behave with respect to their backbone rigidity and, by extension, to residue order and disorder. This is exemplified by the per-amino-acid dynamics properties shown in Fig. 1 . Advances in the way the S 2 values are calculated from the chemical shifts, and inclusion of other types of experimental NMR data (for example, relaxation parameters) additionally have great potential to further improve the conversion of NMR parameters into per-residue dynamics information. These developments, in combination with the now well-established relationship between protein dynamics and function, open up avenues to add a new dimension to the sequence-only analysis of proteins from genomics. This is especially the case for IDPs, where dynamics has a key role in determining their characteristics [34] . The >50 predictors published to date employ many different computational principles but most of them rely on data from DisProt [4] . Despite the recent development of, for example, meta-predictors, improvements in the field are still highly necessary [9] . The physical basis of protein disorder also remains unclear when using these predictors, and we here confirm the suspicion that actual values of the disorder-prediction scores have some direct meaning themselves [19] (see Methods). It is in this context important to position the DynaMine predictions in relation to a previous work [35] that indicates a connection between predicted free energy and disorder; DynaMine predicts dynamics as observed for the proteins in our data set in their energetically favourable states. We show that these energetically favourable dynamics are also physically linked with structural disorder, thus firmly establishing the link between the two. Our approach thus overcomes the key limitations related to the binary treatment of O/D and the source of disorder data; it is rooted in experimental chemical shift data encompassing fast backbone dynamics, uses a continuous scale for expressing backbone movements and avoids the use of 3D structures. Even though especially NMR structures are also a good source of information to train or tune predictors [18] , and structures can be used to predict S 2 values [17] , they do not represent the conformations of the protein in solution for more dynamic regions. Specialist approaches with careful use of experimental data are required in such cases [36] . DynaMine can also pinpoint function-related features in sequences. It defines the boundaries of folded domains and secondary structure elements and seems to be sensitive to different disordered states distinguished by their level of global organization. Structural disorder was roughly classified into two global types [37] : extended (random coil-like) and collapsed (molten globule-type). DynaMine has the ability to outline molten globule regions (for example, NCBD or CBP) embedded in a more disordered structural environment. IDPs often recognize their binding partners via short continuous sequence motifs, which are frequently defined by local sequence conservation [38] , [39] and structural bias towards the bound conformational state [6] , [7] , [8] . DynaMine seems to be capable of picking up locally reduced dynamics in these regions, which appear as peaks in the prediction. For functional motifs that are not supposed to fold up on binding, as in post-translational modification sites and targeting motifs determining subcellular location, peaks are not predicted. In some cases, clear minima even occur that indicate the highly exposed nature of these sites, as in the segment of p53 bound by the ubiquitin ligase USP7 and its nuclear localization signal motifs. DynaMine might therefore provide vital information in correctly identifying and assigning types of functional motifs from sequence, which will be the subject of a future comprehensive analysis of correlations with data in the ELM [40] and MiniMotif [41] databases. Furthermore, the excellent performance of DynaMine suggests that the dynamical characteristics of a residue might be fundamentally encoded in the protein sequence. A recent large-scale in silico study using molecular dynamics simulations from 3D protein structures showed that dynamics and function are closely related [42] and identified dynamics patterns in proteins (the ‘Dynasome’). Although the (experimental) order parameter is related to fast (ps-ns timescale) backbone dynamics, DynaMine shows a strong correlation with observed (binary) structural disorder, which is more related to slower (up to high μs), segmental motions of the polypeptide chain. This excellent agreement probably comes from two distinct, albeit interrelated, sources. First, it has been shown in the literature that fast local motions and slower, segmental motions are tightly linked [15] , where collective fast motions make up larger-scale, slower segmental rearrangements of the polypeptide chain. Second, the chemical-shift-estimated are potentially linked to slower- and larger-scale conformational exchange phenomena such as transition between different secondary structures, as long as these cause averaging of chemical shifts (see Methods). When we predict S 2 from chemical shifts (and sequence), it represents a mixture of fast and slower motions in unknown proportions, which strengthens the physical meaning of the data underlying DynaMine as a disorder predictor. This might also explain why it works so well with a long (51 residue) window. In all, the use of DynaMine opens up the enormous pool of available protein sequences lacking structure information for similar dynamics analysis. It may also give us important clues on diseases, in which the mutations causing critical changes in the structure and/or dynamics of IDPs lead to alterations in function and/or aggregation of the protein [43] , [44] . To conclude, we contend that DynaMine provides independent evidence and an unbiased picture of dynamics and structural disorder. We anticipate that DynaMine will be used for assessing and estimating the stability of various substrates (coil-like, molten globule-like and even pre-molten globule-like) and, more importantly, that it will be developed into a tool to assist the prediction of functional regions. Generation of the DS RCI-S2 data set of values To ensure that the chemical-shift values reflect proteins in physiological conditions, only BMRB entries that fulfil the following criteria were retained: pH between 5.0 and 7.0, temperature between 293.0 and 313.0 K, chemical shift data available for C, H and N atoms, and no sample components present from the list in Supplementary Table S1 . For each unique monomeric protein sequence appearing in the resulting set of BMRB entries, the entry with the most chemical-shift data was selected and read into the CCPN framework [45] . The chemical shifts were re-referenced based on the VASCO procedure [46] in case matching PDB coordinates were available, otherwise PANAV [47] was used. A SHIFTY file exported from the CCPN project was then forwarded to the RCI server ( www.randomcoilindex.com ) and the results were stored locally. Confirming the relationship between and values The RCI software calculates a per-residue RCI score for a given sequence for which chemical shift data are available [21] . This RCI score is zero for highly ordered residues and increases to 0.55 for very dynamic residues. The RCI authors proposed a scaling formula (equation 1) to predict S 2 order parameters ( ) directly from the RCI score: This scaling formula is based on the correlation between the RCI score and the S 2 values derived from short molecular dynamics runs and was validated further on a set of 12 proteins for which experimental S 2 order parameters were available [21] . We compared a list of 53 BMRB entries currently available and containing backbone S 2 order parameters derived from amide nitrogen relaxation against the whole BMRB to find entries with matching sequence, sample and sample conditions as well as extensive chemical-shift assignments. This procedure resulted in the DS EXP-RCI-S2 data set of 16 proteins ( Table 1 , Supplementary Table S2 ) comprising a total of 1,581 amino acids (A (136), C (9), E (133), D (107), G (117), F (57), I (86), H (36), K (117), M (29), L (183), N (67), Q (70), S (86), R (87), T (81), W (19), V (117), Y (44)). One entry (bmr5991) overlaps with the set used in the original RCI validation [21] . This analysis confirmed the findings of Berjanskii et al. [21] that the estimations relate well to the experimentally determined values, with an overall observed Pearson correlation of 0.685 for the DS EXP-RCI-S2 data set ( Supplementary Fig. S9A ). Both and cover mainly fast ps-ns dynamics; however, experimental and prediction errors and the way the values are calculated from the experimental relaxation data [48] will result in differences in the produced values. Of particular interest here is that there are variations in the dynamics range covered, as slower (μs and even higher) motions can be captured by the chemical-shift data; this might account for the lower values at high (slower motions are present and incorporated in the ), as well as the higher values at low (slower motions and conformational preference deviate the chemical shift from the ideal random coil value and increase perceived order). For evaluation of the capacity of values to distinguish between ordered and highly dynamic residues as indicated by the values, ROC curves were generated for different cutoffs applied to the value (different colours in Supplementary Fig. S9B ). Residues with values lower than the cutoff are labelled ‘disordered’, all other residues ‘ordered’. The ROC curve then reflects how well the value performs in reproducing these ‘ordered’ and ‘disordered’ categories for the different cutoffs. The results show that the values are very good at distinguishing between these states for residues that are actually highly dynamic (with values of 0.7 or lower) but that this ability is strongly reduced when residues with values >0.7 and <0.8 are included in the ‘disordered’ category. To produce the ROC curve data in Supplementary Fig. S9B a cutoff ranging from 0.55 to 0.85 in 0.05 steps was applied on the values to convert them into two-state O/D annotations. For each cutoff, an ROC curve was then generated in relation to the predicted data. Propensity of amino acids in relation to order classes We removed short sequence fragments occurring with high frequency (such as present in His tags, see Supplementary Table S3 ) from the main DS RCI-S2 set and divided the resulting 216,456 values into bins, with an S 2 value separation of at least 0.025 and containing at least 7,500 residues each ( Supplementary Table S4 ). The resulting 13 bins contained at least 28 points per amino acid. The propensity for each amino acid for each bin was defined similarly to the approach used in GOR secondary structure prediction [49] , with a self-information difference calculated for each bin and each amino-acid residue type (Equation 2): The information difference is calculated from the number of times a residue R is present in a given bin D ( ), the number of times residue R is present in other bins ( ), the total number of residues in the bin ( ) and the total number of residues in all other bins ( ). We used a base 10 logarithm to generate the values. DynaMine backbone dynamics prediction The DS RCI-S2 data set was divided into two subsets: DS RCI-S2_NO_DP , which excludes sequences with >90% sequence identity with any sequence in any DisProt entry, and DS RCI-S2_DP , containing data for all sequences identical to one in DisProt; these are joined into set DS RCI-S2_UNION_DP ( Table 1 ). The DS RCI_S2_NO_DP data are not biased in amino-acid composition and reflect the SwissProt distribution (see Supplementary Fig. S10 ). It was then used to train DynaMine (see Fig. 3 ) based on the linear regression algorithm in Weka 3.6.9 [50] with default parameters. Different regression models were trained using varying sequence window sizes w ; for example, at w equal to 7 the value of the central amino acid and the amino-acid sequence starting at three amino acids before and ending at three amino acids after the central residue are included as input to the learning algorithm. To ensure that each sequence fragment of length w is included only once in the model training, we constructed distributions for all the fragments of length w in the training set and assigned an value corresponding to the median of the distribution after removal of the outliers (the points falling outside the interquartile range). value distributions with a relative s.e. >25% were discarded. The trained DynaMine predictor then takes as input sequence fragments of size w and provides a prediction for the central element of the fragment (the target residue). We assessed DynaMine performance by a 10-fold cross-validation for each w varying between 5 and 51. In this approach, the DS RCI-S2_NO_DP data set was partitioned into 10 subsamples; each of these was used in turn for testing the model trained on the remaining nine subsamples ( Fig. 2a/b ). We also trained a model on the complete DS RCI-S2_NO_DP data set and tested it by predicting the values for the DS RCI-S2_DP data set ( Fig. 2c/d ). Predictions for N- and C-terminal regions If we define the N- and C-terminal residues as the first and last 25 residues in the sequence (based on the 51 residue window size of the predictor), the distribution in DS RCI-S2_NO_DP of values at the termini ( Supplementary Fig. S11B ) is skewed towards lower values compared with the non-terminal regions ( Supplementary Fig. S11A ). The distribution of the values reflects this bias, although the N- and C-terminal values rather overestimate the values; very few values are <0.4 ( Supplementary Fig. S12 ). The peak of most commonly observed values (around 0.9 for ) in contrast shifts to a lower value for (around 0.8). The DynaMine prediction is based on overall statistics and therefore results in narrower S 2 distributions; the simple linear prediction model exemplifies the relevance of the training data and directly reflects previous studies that identified the N- and C-termini of proteins as more likely to be disordered and dynamic [51] , [52] , with ‘almost all proteins (97%) ha[ving] some disordered residues detected within terminal regions’ [52] . Independent data set The independent data set DS IND _ DP contains DisProt entries not in DS RCI-S2_DP that were annotated by X-ray crystallography, NMR, hydrogen–deuterium exchange and mass spectrometry-based high-resolution hydrogen–deuterium exchange or high relative B-factor. We combined these mostly ‘disorder’ annotations with ‘order’ information from the PDB ( Fig. 3 ); for all sequences that have monomeric NMR structures consisting of an ensemble of models, residues were given an ‘order’ annotation if it was found in helix or beta-strand conformation (as determined by STRIDE [53] ) in all of the models. All residues without annotation were not used in the performance comparisons. ROC curves The DynaMine and best performance point on the ROC curves in Fig. 4a were selected as the closest points to the top left corner of the plot (the ideal performance point: maximum true-positive rate (1) and minimum false-positive rate (0)). The thresholds shown for the different disorder predictors are those reported in the corresponding papers or web-server documentations. Disorder predictors Disorder predictions for ESpritz, IUPRED, PONDR VSL2 and RONN were obtained from the corresponding web servers. FoldIndex [32] does not provide values for the first and the last 25 residues of the input sequence; we used a modified version that provides these values, ensuring that the values for the rest of the sequence are identical with those provided by the original FoldIndex. PrDOS2 is the advanced version of the PrDOS disorder-prediction method [29] and takes the evolutionary conservation of the input sequence into account. It is not yet publicly available and we obtained the prediction results directly from the inventor of the method. Relating disorder prediction to values We also addressed the relevance of dynamics and disorder predictions in the context of values. The DS EXP-S2 set contains 22 proteins for which experimental S 2 order parameter values are available, excluding DS RCI-S2 sequences ( Supplementary Table S5 ). We subtracted the values produced by the disorder predictors from 1.0 to obtain values matching the S 2 scale (from 0 to 1), except for FoldIndex where values were used as they are. Supplementary Figure S13A shows the linear correlation and RMSE between the per-residue predictions and values. DynaMine and the Espritz X-ray and NMR predictors give the best results. The reasonable agreement generated by the Espritz predictors confirms previous findings about the capacity of disorder predictors to relate to dynamics [19] . However, all entries in the DS EXP-S2 set have closely related structural entries in the PDB. The Espritz approaches likely include information on these structures, and <15% of the S 2 values DS EXP-S2 contains are <0.8, mostly indicating loops in globular structures. Although the data set does, therefore, not represent intermediate dynamics and disorder well, it is still useful to compare the predictors to the values using a two-state ‘rigid’/‘highly dynamic’ distinction similar to order/disorder, as this is a relative comparison and allows a different examination of their performances in relation to dynamics. Supplementary Figure S13B shows the AUC of the ROC curve for the predictors using different cutoffs to distinguish between ‘highly dynamic’ and ‘rigid’ residues. Higher values indicate better predictions; the predictive capacity of all predictors strongly decreases with increasing cutoff, except for Espritz_DisProt and FoldIndex. The PrDOS2 predictor gives the best performance (although not in an absolute sense, see Supplementary Fig. S13A ); this demonstrates the close connection between disorder and dynamics. The next best results come from DynaMine and the Espritz X-ray and NMR predictors. The relation between the disorder values produced by these best disorder predictors and the actual backbone dynamics of protein residues is evident from this analysis; it solidifies the conclusion that dynamics and disorder are closely connected. Influence of disordered fragment length on prediction accuracy We first compared the content of DS RCI-S2 to the DisProt database (release 6) in terms of disordered fragment length. The lengths of the highly dynamic fragments in the DS RCI-S2 data set (defined as continuous residues with values <0.795) tend to be shorter than the length of disordered fragments annotated in DisProt ( Supplementary Fig. S14 ). We then investigated the influence of the disordered fragment length on the prediction accuracy by subdividing the DS IND_DP into subgroups of short (<20 amino acids), long (between 20 and 50 amino acids) and extremely long (>50 amino acids) fragments, and re-ran the ROC curve analysis as described in Fig. 4b ( Supplementary Fig. S15 ). The DynaMine prediction accuracy for the long and extremely long fragments is comparable to the best predictors, whereas on the short fragments it does better than most. Comparing DynaMine predictions to hydrophobicity scales To ensure that DynaMine does not only reflect hydrophobicity, we performed an analysis of 22 hydrophobicity scales using a 15-residue window with no scaling for the sequences in DS IND_DP . Some of the hydrophobicity-based predictors indeed perform excellently with respect to disorder ( Supplementary Fig. S16 ), although DynaMine outperforms them. DynaMine is, however, a fast backbone dynamics predictor, and we also compared the hydrophobicity predictions against the values. To normalize the hydrophobicity values, we first applied a normalization function to obtain hydrophobicity values ranging from the lowest and highest values and reversed the hydrophobicity values in case of negative linear correlation so as to obtain the lowest RMSE. The results of this analysis are shown in Supplementary Fig. S17 (similar to Supplementary Fig. S13A ), and they show that hydrophobicity alone does not reflect the values at all. This demonstrates that the DynaMine predictions go well beyond what traditional hydrophobicity scales can provide. DynaMine availability The DynaMine predictor model file to be used within the Weka framework is available upon request from the authors. The Weka command line can be used to get the DynaMine predictions in the following way: java classpath weka.jar weka.classifiers.functions.LinearRegression -T <the input sequence in ARFF format> -l <the DynaMine model file> -p 1-51 An example of input sequence (for p53) in the ARFF format (command line option -T) compatible with the DynaMine predictor is provided as Supplementary Data 1 (dataset.arff). We also provide as Supplementary Software 1 a wrapper python script (wrapper_predict.py) that can take a FASTA file as input, to be launched as follows. python wrapper_predict.py myProtein.fasta In the Supplementary Software 2 (config.py) the javacmd variable should be modified to the system requirements. The wrapper_predict.py script produces the input for the Weka framework and manages the Weka output through two python scripts ( Supplementary Software 3 , produce_input.py and Supplementary Software 4 , print_predictions.py) with BioPython dependencies. How to cite this article: Cilia, E. et al. From protein sequence to dynamics and disorder with DynaMine. Nat. Commun. 4:2741 doi: 10.1038/ncomms3741 (2013).